Crustaceans from bitumen clast in Carboniferous glacial diamictite extend fossil record of copepods Copepod crustaceans are extremely abundant but, because of their small size and fragility, they fossilize poorly. Their fossil record consists of one Cretaceous (c. 115 Ma) parasite and a few Miocene (c. 14 Ma) fossils. In this paper, we describe abundant crustacean fragments, including copepods, from a single bitumen clast in a glacial diamictite of late Carboniferous age (c. 303 Ma) from eastern Oman. Geochemistry identifies the source of the bitumen as an oilfield some 100–300 km to the southwest, which is consistent with an ice flow direction from glacial striae. The bitumen likely originated as an oil seep into a subglacial lake. This find extends the fossil record of copepods by some 188 Ma, and of free-living forms by 289 Ma. The copepods include evidence of the extant family Canthocamptidae, believed to have colonized fresh water in Pangaea during Carboniferous times. No group of Metazoa exhibits the range of morphological diversity as observed among Crustacea [1] , and this structural disparity is best demonstrated by the ubiquitous Copepoda. Copepods outnumber every other group of multicellular animals on Earth, including the hyperabundant insects and nematode worms [2] , [3] . These small crustaceans are found throughout the world's natural and man-made aquatic environments, spanning the entire salinity range from fresh water to hypersaline, and a vertical range that extends from the nutrient-rich black oozes of the oceanic abyss [4] down to 10,000 m to the oligotrophic waters at 5,500 m altitude in the Himalayan mountains [5] . With more than 12,500 species, and outnumbering insects in abundance by up to three orders of magnitude [6] , copepods carry a global biological importance. Current evidence suggests that copepods originated in the marine hyperbenthic environment [3] and subsequently colonized the entire salinity spectrum, with major habitat shifts into the marine plankton and continental fresh waters. In terms of speciation and adaptive radiation, one of the most extraordinary aspects of the Copepoda is their capacity to enter into associations with other organisms [7] , [8] . Copepod symbionts display the highest taxonomic range of associates and hosts of any extant metazoan group; perhaps no other taxon has been so adaptable in host utilization. Nearly half of all known copepod species (approximately 4,300 species in 109 families) are symbionts, using hosts from almost every aquatic animal phylum, from sponges to mammals and reptiles. A crude estimate based on morphology suggests that there have been 11 or more independent origins for symbiosis across the various copepod orders, with a minimum of seven independent colonization events in fish. Among chordates, parasitic copepods are found across the entire vertebrate size spectrum, from the magnificent blue whale, Balaenoptera musculus [9] , to the smallest extant fish species, Paedocypris progenetica [10] (see also R.H., unpublished data). As a group, copepods exhibit an unusually diverse range of body forms, live in every conceivable environment (except aerial), and display a wide variety of life history modes, as predators, herbivores and parasites. However, their global dominance and diversity is only part of their success story. Copepods underpin the world's freshwater and marine ecosystems, having a major role in aquatic foodwebs [11] . They are sensitive bioindicators of local and global climate change [12] , key ecosystem service providers [13] , [14] and parasites of economically important aquatic animals, being responsible for disease-related fish losses that exceed 430 million USD worldwide per annum [15] . Copepods sustain the majority of world fisheries [11] , and through their roles as vectors of disease [16] , [17] also have a number of direct and indirect effects on human health and quality of life. Despite their long evolutionary history, few fossil-based calibration points are available that could provide insights into the divergence times of the various copepod lineages and the origin of their major radiation events. Copepods are typically minute and fragile; hence they have low fossilization potential and their body fossil record consists principally of one Cretaceous parasite [18] , [19] and some Miocene fossils [20] . Here, we report a unique occurrence of copepod and other crustacean fragments preserved in a single bitumen clast from a glacial diamictite of Carboniferous age from Oman, which extends the fossil record of copepods back by some 188 Ma, and of free-living forms by 289 Ma. Geochemical analyses indicate that the source was probably a bitumen seep some 100–300 km southwest of the present position of the diamictite, which concurs with geological evidence of ice flow direction. Pollen in the diamictite indicates a late Carboniferous age, but the lack of palynomorphs in the clast suggests that the bitumen is the result of an oil seep into a subglacial lake with no open water. Some of the fragments seem to belong to the harpacticoid copepod family Canthocamptidae, the members of which typically inhabit fresh waters (including glacial lakes) today [21] . This record concurs with suggestions that harpacticoid copepods colonized fresh waters during the assembly of Pangaea [22] . However, the circumstances of the discovery mean that bitumen in diamictite is unlikely to be sufficiently common to be a productive source of fossil crustaceans in the future. Geology The clast of solid bitumen (pitch; Fig. 1a ) was discovered during a field excursion to outcrops of the Permo-Carboniferous glacial Al Khlata Formation deposits in the Huqf Outcrop area of eastern interior Oman in January 2004. The solitary clast was located within a massive diamictite (Global Positioning System location: 19° 45′ 59.2″ N, 57° 26′ 14.9″ E, Fig. 1b ) of the Al Khlata Formation ( Fig. 1d ), which exhibits vertically oriented clasts and clast clusters, and passes up without sedimentary break into a stratified diamictite, thus showing the features of deposition from a subglacial rain-out or melt-out [23] . The diamictite overlies a well-known Al Khlata Formation striated pavement located 260 m east–southeast of the bitumen-clast locality [24] , [25] . Palynological assemblages recovered from the diamictite contain no marine palynomorphs. Spores and pollen, including Anapiculatisporites concinnus , Potonieisporites spp. and Punctatisporites spp., indicate that it is late Carboniferous in age (Westphalian–Stephanian; early P5 or OSPZ1 [26] , [27] ). The bitumen clast is of pebble size, angular to subrounded, with a slightly weathered, dull exterior and a microfractured shiny interior ( Fig. 1a ). Despite intensive searching, no further bitumen clasts have been found in this diamictite nor others in the Al Khlata outcrop area. 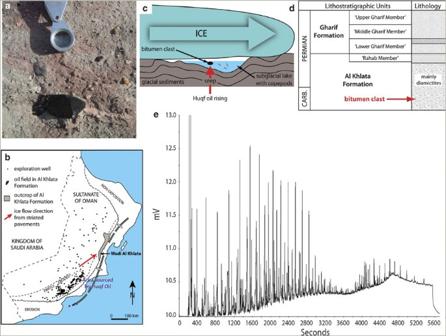Figure 1: Geological setting of the bitumen clast in the Al Khlata Formation, upper Carboniferous, Oman. (a) The bitumen clastin situin Al Khlata Formation diamictite. (b) Location map of the Sultanate of Oman showing the bitumen clast locality (Wadi Al Khlata) in relation to the outcrop and subsurface extent of the Al Khlata, the likely source of the bitumen in the Thuraya area, and the ice flow direction as evidenced by glacially striated pavements. (c) Diagram showing our interpretation of the origin of the bitumen clast and its crustacean fragments. (d) Stratigraphy of the Al Khlata Formation showing the relative age of the deposits containing the bitumen clast. (e) Gas chromatogram of the solvent-soluble fraction of the bitumen clast. The chromatogram is unusual for a surface petroleum sample, as it contains a series of apparently unalteredn-alkanes in the range of nC7 to nC27. Biodegradation of surface oil seeps normally removes some or all of then-alkanes present60. The relatively high abundance of biomarker compounds eluting between 4,000 and 5,000 s is indicative of mixing of at least two oil charges from Huqf source rocks. Thermal maturity of the bitumen, estimated from molecular distributions of biomarker compounds and from bitumen reflectance analysis, suggests relatively low thermal maturity of the high-molecular-weight fraction (equivalent approximately 0.6% vitrinite reflectance). Figure 1: Geological setting of the bitumen clast in the Al Khlata Formation, upper Carboniferous, Oman. ( a ) The bitumen clast in situ in Al Khlata Formation diamictite. ( b ) Location map of the Sultanate of Oman showing the bitumen clast locality (Wadi Al Khlata) in relation to the outcrop and subsurface extent of the Al Khlata, the likely source of the bitumen in the Thuraya area, and the ice flow direction as evidenced by glacially striated pavements. ( c ) Diagram showing our interpretation of the origin of the bitumen clast and its crustacean fragments. ( d ) Stratigraphy of the Al Khlata Formation showing the relative age of the deposits containing the bitumen clast. ( e ) Gas chromatogram of the solvent-soluble fraction of the bitumen clast. The chromatogram is unusual for a surface petroleum sample, as it contains a series of apparently unaltered n -alkanes in the range of nC7 to nC27. Biodegradation of surface oil seeps normally removes some or all of the n -alkanes present [60] . The relatively high abundance of biomarker compounds eluting between 4,000 and 5,000 s is indicative of mixing of at least two oil charges from Huqf source rocks. Thermal maturity of the bitumen, estimated from molecular distributions of biomarker compounds and from bitumen reflectance analysis, suggests relatively low thermal maturity of the high-molecular-weight fraction (equivalent approximately 0.6% vitrinite reflectance). Full size image Organic geochemical analyses on the bulk bitumen indicate that it is homogeneous, with small microcracks and inclusions of mineral matter. Molecular and carbon isotope analyses were carried out on fluid extracted from the sample by dichloromethane. The whole-extract gas chromatogram ( Fig. 1e ) is unusual in showing no evidence of the removal of n-alkanes in the range of nC7 to nC27. Biodegradation of surface oil seeps normally removes some or all of the n-alkanes present. Biomarker and carbon-isotope analyses indicate a mixed source for the bitumen from pre- and intra-salt Huqf source rocks of infra-Cambrian age, with no evidence of a contribution from Q oil sources [28] . The bitumen clast is thus similar to oils that occur today on the eastern flank of the South Oman Salt Basin 100–300 km to the southwest ( Fig. 1b ); therefore, it must have undergone transport, presumably by glacial processes, from the eastern flank area to the Huqf area during late Carboniferous times, which is supported by the ice flow direction preserved on Oman glaciated pavements. As the bitumen clast occurred within an upper Carboniferous diamictite, the clast and the organic material it contains must be at least late Carboniferous in age. The possibility that the clast is older and was reworked into upper Carboniferous glacial deposits cannot be ruled out; however, this seems unlikely given the relatively low mechanical strength of solid bitumen and the relatively large size of the Al Khlata clast. Because the bitumen is from a Huqf source that was already mature at this time [28] , [29] , and because it occurs within a rain-out diamictite with no evidence of marine influence, it seems likely that it reached the surface subaqueously in a subglacial lake. In the area of the likely oil seepage, glacial lake sediments of the same P5 age as that which contains the bitumen clast directly overlie Devonian sands and shales. Because of the low density of the warm oil, it rose through the cool water column as a globule, presumably engulfing and entombing the crustaceans as it ascended ( Fig. 1c ). This sequence of events would explain the lack of pollen and spores in the bitumen as these would be rare in a subglacial lake in which ice cover would have prevented spores and pollen from reaching the lake waters. The fragmented nature of the fossils may relate to their inclusion in the warm oil globule that broke them up as it ascended and solidified into pitch. Palaeontology The organic residue after maceration of the bitumen consists of dark brown, resinous material immediately recognizable as crustacean remains, no palynomorphs and little other organic material, apart from amorphous organic fragments. The arthropod remains consist of thousands of fragments ranging from 50 to 250 μm in size ( Figs 2a–i and 3a–g ). The fragments are referred to as Crustacea on account of their biramous appendages, setae with setules and freshwater origin. There are no whole specimens, no body parts and very few trunk appendages; nearly all are cephalic appendage fragments, including antennulary and antennary segments, mandibular gnathobases and maxillary endites. Preservation is exceptional in that some fragments show muscles ( Fig. 2e ), jointed setae ( Figs 2h,i ), geniculate setae ( Figs 2h,i ) and spinular ornamentation ( Fig. 3b ). The possibility of contamination with recent crustaceans can be ruled out because the preparation included repeated washing of the unprocessed clast so that nothing is adhered to the surface, and bitumen pieces from the centre of the clast were processed, which would not have been exposed since Carboniferous times. 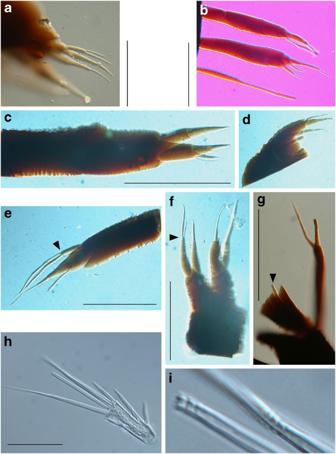Figure 2: Crustacean fragments from upper Carboniferous bitumen clast. (a) Endopod of a maxilla, possibly of copepod. (b) Endites of crustacean maxilla. (c) Distal segment of exopod of biramous trunk limb (seeFigure 3a). (d) Fragment of crustacean maxilla or maxilliped. (e) Maxillary endite with jointed elements (arrowed). (f) Pair of maxillary endites, joint arrowed, of possible copepod. (g) A part of maxilla; arrow points to intrinsic muscle showing strands. (h) Distal part of antennary endopod of canthocamptid copepod. (i) Detail of geniculate setae ofh. Scale bars, 50 μm. Figure 2: Crustacean fragments from upper Carboniferous bitumen clast. ( a ) Endopod of a maxilla, possibly of copepod. ( b ) Endites of crustacean maxilla. 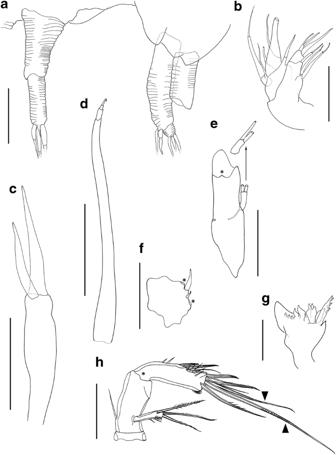Figure 3: Crustacean fragments from upper Carboniferous bitumen clast. (a) Unknown crustacean: pair of biramous trunk limbs showing two-segmented rami; endopod on left side missing; exopod incomplete on right side; note incomplete annulations. (b) Maxilla of possible copepod. (c) Large appendage fragment, possibly an endite, of unknown crustacean. (d) Large appendage fragment of uniramous trunk limb with curved claw. (e) Allobasis of antenna (insert showing exopod) of canthocamptid copepod; asterisk indicates condyle. (f) Antennulary segment of copepod; asterisks indicate insertion scars of missing armature elements. (g) Mandibular gnathobase of copepod. (h) Modern canthocamptid antenna: explanatory key forFigures 2h, iand3e; asterisk indicates condyle, geniculations arrowed. Scale bars, 100 μm (c,d), 50 μm (a,b,e,f,h), 25 μm (g). ( c ) Distal segment of exopod of biramous trunk limb (see Figure 3a ). ( d ) Fragment of crustacean maxilla or maxilliped. ( e ) Maxillary endite with jointed elements (arrowed). ( f ) Pair of maxillary endites, joint arrowed, of possible copepod. ( g ) A part of maxilla; arrow points to intrinsic muscle showing strands. ( h ) Distal part of antennary endopod of canthocamptid copepod. ( i ) Detail of geniculate setae of h . Scale bars, 50 μm. Full size image Figure 3: Crustacean fragments from upper Carboniferous bitumen clast. ( a ) Unknown crustacean: pair of biramous trunk limbs showing two-segmented rami; endopod on left side missing; exopod incomplete on right side; note incomplete annulations. ( b ) Maxilla of possible copepod. ( c ) Large appendage fragment, possibly an endite, of unknown crustacean. ( d ) Large appendage fragment of uniramous trunk limb with curved claw. ( e ) Allobasis of antenna (insert showing exopod) of canthocamptid copepod; asterisk indicates condyle. ( f ) Antennulary segment of copepod; asterisks indicate insertion scars of missing armature elements. ( g ) Mandibular gnathobase of copepod. ( h ) Modern canthocamptid antenna: explanatory key for Figures 2h, i and 3e ; asterisk indicates condyle, geniculations arrowed. Scale bars, 100 μm ( c , d ), 50 μm ( a , b , e , f , h ), 25 μm ( g ). Full size image Although many of the fragments that we refer to as indeterminate Crustacea ( Figs 2b–f and 3a,c,d ) can be excluded from the Copepoda, a few of the crustacean remains can be assigned with confidence to that group. Although unique autapomorphies (for example, intercoxal sclerite, presence of a first copepodid stage in the life cycle) of the subclass Copepoda are few [3] and not seen in our fragmentary material, various lines of evidence point not only to Copepoda but also to ordinal and familial ranks within the subclass. Evidence for copepods comes from the size of the fragments, geniculate setae (displaying a well-defined flexure zone) on the antennary endopod ( Figs 2h,i , cf. 3h) and the characteristic condyle between the allobasis and the endopod of the antenna ( Fig. 3e ). The size and structure of the mandibular gnathobase ( Fig. 3g ) also indicate a copepod origin. The combination of geniculate setae on the antennary endopod and the presence of an exopod on the allobasis place some of the copepod remains in the order Harpacticoida, and specifically the family Canthocamptidae. Geniculate setae have been observed on the branchiostegites of some decapod crustaceans [30] and on the prodorsum and hypostome of certain acarid mites [31] , [32] but their location and morphology are clearly different. Copepods dominate the holozooplankton community in the largest biome on Earth—the 1,347,000,000 km 3 of the open pelagic water column—and also live in virtually all freshwater habitats [33] and as symbionts of invertebrate and vertebrate hosts [7] , [8] . Approximately 2,814 species live in continental habitats, from the largest ancient lakes to subterranean waters, from glacial pools [34] to hot springs, and from hypersaline lakes to phytotelmata [35] . There is overwhelming evidence that the ancestors of modern freshwater copepods evolved in marine environments, where they existed and diversified over millions of years [3] . At least 22 independent colonizations of fresh and inland continental waters have been identified [22] , 10 of which represent harpacticoid lineages. The timing of colonization events has been estimated by inference from biogeographical data, and it was suggested that there was a succession of at least four major waves of colonization of inland continental waters by harpacticoids. On the basis of its modern cosmopolitan distribution, the Canthocamptidae (600+ spp.) has been claimed to be in the first wave of copepod colonization of the whole of Pangaea around 250 Ma [22] . This suggestion is in accordance with the present finding of freshwater copepod remains. The fossil record of copepods is meagre, consisting of a subfossil harpacticoid from a Neolithic cave floor in Kent, United Kingdom [36] , a Pleistocene harpacticoid from a lake deposit in Argentina [37] , a cyclopoid and the harpacticoid Cletocamptus sp. from a Miocene lake deposit in California [20] and a fish parasite from the Cretaceous Santana Formation of Brazil, currently referred to the extant siphonostomatoid family Dichelesthiidae [19] . Possible Cretaceous amber copepods were reported from Canada [38] and Spain [39] , but both specimens are mere ghostly shapes, and the former could not be traced in the collections. A possible copepod or remipedian affinity was put forward for a fossil from the lowermost Ordovician of Öland, Sweden, although without much evidence or confidence [40] . Until now there have been no records of copepods from ancient bitumen, although other crustaceans are well known to have come from bitumen, particularly from Tertiary and younger deposits [41] . Subfossil copepod eggs have been reported from Quaternary sites [42] , [43] , and it is thought that some Phanerozoic acritarchs may be copepod eggs [44] , [45] , [46] . Fossil galls resulting from the activities of parasitic copepods were reported from Middle and Late Jurassic echinoderms [47] . Thus, body-fossil and trace-fossil evidence places the previously oldest known Copepoda to early Cretaceous or early Jurassic, respectively, but the fossil fragments reported here indicate that modern copepods have existed since at least late Carboniferous times. The phylogenetic consensus tree ( Fig. 4 ) is based on morphology [1] and recently obtained results derived from small subunit ribosomal DNA (18S) sequence data [48] and show the effect of the new find on the geological history of copepods. The new evidence not only takes the fossil record of Harpacticoida back to Carboniferous times but also that of the primarily planktonic but more primitive orders Platycopioida, Calanoida and Mormonilloida. The monophyly of Copepoda is generally accepted [3] , [49] , [50] , but their relationship with other groups within the Crustacea has been contentious. Copepods have traditionally been placed in the heterogeneous class Maxillopoda, which seems to be an assemblage of short-bodied taxa with morphological characteristics, such as gonopore location or nauplius eye structure, which link together different combinations of subgroups [1] . Some morphological studies [51] , [52] have recognized two lineages within the Maxillopoda and placed the Copepoda, Mystacocarida and the extinct Skaracarida in the copepodan lineage as sister to the thecostracan lineage; however, there is now a general consensus that there is neither robust morphological [1] , [53] nor molecular [54] , [55] , [56] , [57] support for maxillopodan monophyly. A recent phylogenomic analysis [58] of 62 nuclear protein-coding sequences revealed an unanticipated group (Multicrustacea or 'numerous crustaceans') embracing the Copepoda as sister to a thecostracan-malacostracan clade. Bayesian statistical (non-clock) estimates of divergence times [54] suggest that thecostracans (barnacles and relatives) and malacostracans (crabs and relatives) separated no later than 459 Ma (Middle Ordovician). The basal divergence of the Copepoda within the Multicrustacea must therefore have occurred much earlier but conceivably not before the emergence of the Branchiopoda (the sistergroup of the Multicrustacea [58] ) at 521 Ma [54] . Our new material conclusively extends the copepod fossil record back to the late Carboniferous period, but extrapolation of available divergence dates suggests that the most abundant pancrustacean clade had already originated in the Cambrian. 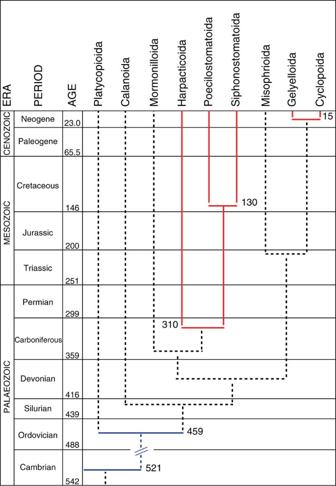Figure 4: Phylogenetic tree of the Copepoda. The consensus cladogram based on morphology3and small subunit ribosomal DNA sequence data48is superimposed on the geological column and shows the known body fossil record of copepods (red lines), as well as the predicted origin of the group (blue lines). Figure 4: Phylogenetic tree of the Copepoda. The consensus cladogram based on morphology [3] and small subunit ribosomal DNA sequence data [48] is superimposed on the geological column and shows the known body fossil record of copepods (red lines), as well as the predicted origin of the group (blue lines). Full size image Bitumen is a rare but effective hosting medium for Fossil-Lagerstätten, best known in oil sands and tar pits such as La Brea, California [59] ; however, the discovery reported here is the first record of preservation of fossil soft parts in an isolated bitumen clast. The preservation of crustacean fragments is exceptional, including muscle fibres ( Fig. 2g ), which, together with the lack of degradation shown by the bitumen in this study, is remarkable. This suggests the need for further study of the taphonomy of crustacean cuticles, using pyrolysis gas chromatography, for example, should more such clasts come to light. Palynology In an attempt to understand more about its age and origin, and with the possibility that it might contain trapped biota, parts of the clast were prepared for palynology and organic geochemistry. The material was broken up to approximately pea-sized pieces, and each piece subjected to a different process, including dissolution, using very strong solvents, assisted by heat. Solvents and methods attempted on separate samples of bitumen included 100% dichloromethane and ultrasonication (for 30 min); 50:50 of dichloromethane/methanol and ultrasonication (for 30 min); 100% dimethylsulphoxide (for 2 weeks); 30% hydrogen peroxide (for 4 days); and 50:50 of 30% hydrogen peroxide/concentrated nitric acid (for 4 days). Such attempts at liberation by simple dissolution were unsuccessful, the bitumen being almost completely insoluble to most solvents. The most successful method of liberation was long periods (12–24 h) of oxidation by Schultze's Solution and/or fuming nitric acid, and then treatment with a 5% potassium hydroxide solution. With both acids, the solid bitumen was reduced to a solution, which could be poured off, leaving a residue of solid, fine organic residue. Enough organic residue from a small piece of solid bitumen was released to allow several microscope slide preparations to be made. Geochemistry Molecular and carbon isotope analyses were carried out on bitumen extracted from the solid sample by dichloromethane. The solvent extractable organic matter from the sample was fractionated into saturated and aromatic hydrocarbon fractions by MPLC. The hydrocarbon fractions were analysed by gas chromatography–mass spectrometry to determine their biomarker compositions. Bulk hydrocarbon isotope values were measured on saturated and aromatic hydrocarbon fractions. Compound-specific carbon isotope analyses were carried out on the alkane fraction that was separated from the saturated hydrocarbons of the bitumen extract using a molecular sieve technique. Palaeontology Arthropod fragments were cleared in 90% lactic acid for 2 weeks and subsequently mounted on slides in lactophenol mounting medium. Some fragments (for example, Fig. 2h,i ) were carefully warmed in 10% KOH by weight in distilled water at about 90 °C for 12 h and this procedure was repeated in 90% lactic acid to reveal additional detail. Glass fibres were added to prevent distortion of the length/width ratios and of the three-dimensional structure of the appendages and to facilitate rotation and manipulation, allowing observation from all angles. Preparations were sealed with transparent nail varnish. All drawings have been prepared using a camera lucida on a Leica DMR differential interference contrast microscope. Measurements were taken with an ocular micrometre. The material is deposited in the collections of the Department of Zoology, Natural History Museum, London. How to cite this article: Selden, P.A. et al . Crustaceans from bitumen clast in Carboniferous glacial diamictite extend fossil record of copepods. Nat. Commun. 1:50 doi: 10.1038/ncomms1049 (2010).